Spatial control of defect creation in graphene at the nanoscale Defects in graphene alter its electrical, chemical, magnetic and mechanical properties. The intentional creation of defects in graphene offers a means for engineering its properties. Techniques such as ion irradiation intentionally induce atomic defects in graphene, for example, divacancies, but these defects are randomly scattered over large distances. Control of defect formation with nanoscale precision remains a significant challenge. Here we show control over both the location and average complexity of defect formation in graphene by tailoring its exposure to a focussed electron beam. Divacancies and larger disordered structures are produced within a 10 × 10 nm 2 region of graphene and imaged after creation using an aberration-corrected transmission electron microscope. Some of the created defects were stable, whereas others relaxed to simpler structures through bond rotations and surface adatom incorporation. These results are important for the utilization of atomic defects in graphene-based research. Defects in graphene [1] not only modify its properties [2] , [3] , [4] , [5] , [6] , [7] , [8] , [9] , [10] , [11] but also extend its functionality by providing sites for chemical reactions, which enables intentional doping at specific points. Electron and ion beam irradiation have been successful in generating defects in carbon nanostructures, such as fullerenes, nanotubes, peapods, and recently graphene [12] , [13] , [14] , [15] , [16] , [17] , [18] , [19] , [20] , [21] , [22] , [23] . For ion beam irradiation, defects are sporadically formed over a wide area of graphene with lack of nanoscale spatial control and in situ monitoring at the atomic level. Alternatively, electron beam irradiation within an aberration-corrected transmission electron microscope (AC-TEM) allows in situ atomic level monitoring without having to remove the sample from vacuum or subject it to further characterization methods. Electron beam irradiation of graphene well above its knock-on damage (KOD) threshold of ∼ 86 keV within an AC-TEM generates defects that can be subsequently imaged, with the electron beam accelerating voltage reduced to below the KOD threshold after defect creation to minimize further beam damage [19] , [20] , [21] , [22] , [23] . However, this approach exposes a large amount of the graphene to electrons with energy above the KOD threshold, and limiting defect creation to one specific location is nearly impossible. Efforts to control defect creation in graphene within a specified nanoscale region using a focussed electron beam in a TEM have been limited to the creation of nano-pores or small holes in the graphene [24] , [25] . In this case the energy of the electron beam was above the KOD threshold and it is likely that many other wide-spread smaller vacancies are also formed throughout the graphene sample. Scanning transmission electron microscopy (STEM) has also been used to create vacancies in a carbon nanotube by the use of an intensely focussed electron beam above the KOD threshold, but again it is likely that many other smaller defects such as monovacancies were also created within the sample [26] . A key challenge in this area of graphene research is the ability to induce defects only within the specified area of interest and then be able to image the structure without creating further defects. We address this challenge and demonstrate nanoscale control of defect creation in monolayer chemical vapour deposition (CVD) graphene with minimal contamination. The electron beam irradiation potential is set to 80 kV within an AC-TEM, which is just below graphene's theoretical KOD threshold. However, we reveal that substantially increasing the electron beam current density (BCD) results in localized sputtering of graphene, even below the KOD threshold of 80 kV. We show that by careful control of the electron BCD, defect creation can be confined to within a 10×10 nm 2 region of graphene and the average level of complexity controlled by the exposure time. 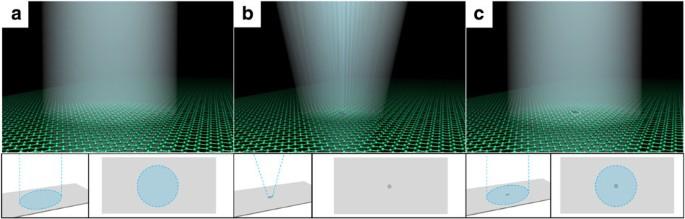Figure 1: Creating defects with an electron beam. Schematic illustrating the beam profile used in the three principle stages: (a) a broad beam used to image graphene before defect formation (typical beam current density∼105e−1nm−2s−1), (b) a focussed probe with a high current density used to form defects (∼108e−1nm−2s−1) and (c) a broad beam used to image graphene after defect formation (∼105e−1nm−2s−1). Controllable defect creation Figure 1 illustrates the concept of our nanoscale control of defect creation; the beam is set to normal imaging conditions with uniform illumination at a BCD ∼ 10 5 e −1 nm −2 s −1 ( Fig. 1a ). No defects in graphene were created under these conditions, consistent with previous reports [19] , [20] , [21] , [22] , [23] . A reference image is taken of the pristine graphene lattice. Next the beam is focussed to a BCD ∼ 10 8 e − 1 nm −2 s −1 within a 10-nm diameter spot to create defects ( Fig. 1b ). The exposure time is varied as desired and then the beam is expanded back to the original conditions for imaging ( Fig. 1c ) and an image is taken of the created defects, typically within 30–60 s. This delay was due to the need to readjust the focus and twofold astigmatism. Figure 1: Creating defects with an electron beam. Schematic illustrating the beam profile used in the three principle stages: ( a ) a broad beam used to image graphene before defect formation (typical beam current density ∼ 10 5 e − 1 nm −2 s −1 ), ( b ) a focussed probe with a high current density used to form defects ( ∼ 10 8 e − 1 nm −2 s −1 ) and ( c ) a broad beam used to image graphene after defect formation ( ∼ 10 5 e − 1 nm −2 s −1 ). Full size image Defects were created in a clean area of pristine graphene only when the BCD reached ∼ 10 8 e − 1 nm −2 s −1 . Analysis of the spatial profile of the electron beam showed a non-uniform BCD when focussed, with over half the total beam current contained within a zone of ∼ 10 nm diameter ( Supplementary Fig. S1 ). It is within this 10 nm hot spot that the BCD reaches 10 8 e − 1 nm −2 s −1 and results in the created defects being confined to this region. After focussing the probe, a predetermined time was allowed to elapse before the beam was defocused to image the specimen. Manipulating the exposure time to the focussed beam gives a degree of control over the average complexity of the defects that are formed, as demonstrated in Figs 2 and 3 . 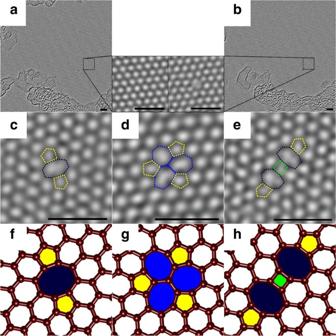Figure 2:Formation of defects after a 30 s electron beam exposure. (a) AC-TEM image of a pristine graphene sheet before 30 s exposure to a focussed electron beam. (b) Divacancy formed in exposure area directly after irradiation. Inserts show magnified images of highlighted areas ina,b. AC-TEM images of three different 30 s exposures, resulting in (c) a divacancy, (d) a divacancy having undergone a single Stone-Wales bond rotation and (e) two linked divacancies along the armchair direction. (f–h) Atomic models corresponding to the TEM images inc–e, respectively. The colour scheme (dashed line annotations and model filling colour) denotes the number of carbons in the respective carbon ring, such that green, yellow, blue and dark blue represent 4-, 5-, 7- and 8-membered carbon rings, respectively. Non-annotated images are presented inSupplementary Fig. S2. Scale bars represent 1 nm. Figure 2a shows an AC-TEM image of a pristine graphene sheet before a 30-s exposure, Fig. 2b directly after, with a single divacancy in the exposed area. AC-TEM images from three 30-s exposures in different pristine regions are shown in Fig. 2c–e . The divacancy structures observed have two adjacent atoms removed from the lattice, and in the case of Fig. 2d the divacancy has undergone a single Stone-Wales (SW) transformation [27] . In Fig. 2e two divacancy defects are joined, forming an extended defect along the armchair lattice direction (see Supplementary Fig. S3 ). Monovacancies were observed less frequently due to the high energy of the monovacancy configuration, which leaves one carbon atom in an unsaturated state with only two bonds, and is thus unstable with respect to the more energetically favourable divacancy structure when under electron beam irradiation [21] . Figure 2: Formation of defects after a 30 s electron beam exposure . ( a ) AC-TEM image of a pristine graphene sheet before 30 s exposure to a focussed electron beam. ( b ) Divacancy formed in exposure area directly after irradiation. Inserts show magnified images of highlighted areas in a , b . AC-TEM images of three different 30 s exposures, resulting in ( c ) a divacancy, ( d ) a divacancy having undergone a single Stone-Wales bond rotation and ( e ) two linked divacancies along the armchair direction. ( f – h ) Atomic models corresponding to the TEM images in c – e , respectively. The colour scheme (dashed line annotations and model filling colour) denotes the number of carbons in the respective carbon ring, such that green, yellow, blue and dark blue represent 4-, 5-, 7- and 8-membered carbon rings, respectively. Non-annotated images are presented in Supplementary Fig. S2 . Scale bars represent 1 nm. 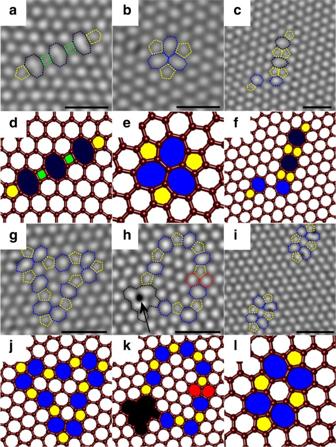Figure 3: Defects created after 60 and 120 s exposures to the electron beam. (a–c) Annotated AC-TEM images of defects formed after 60 s of focussed electron beam irradiation. (a) Three linked divacancies. (b) A divacancy after a SW transformation. (c) Defects clustered around one of a pair of dislocations. Non-annotated images are presented inSupplementary Fig. S4. (d–f) Atomic models of the defects presented ina–c, respectively. (g–i) Annotated AC-TEM images of defects formed after 120 s of focussed electron beam irradiation. (g) An enclosed, rotationally misaligned core of six hexagons, surrounded by a complete loop of pentagons and heptagons. (h) A larger, partially completed loop, isolating several rotated hexagons. A gap in the loop, filled by two hexagonal rings, is highlighted in red. The arrow marks an adatom, which inhibits direct interpretation of the area bordered in black due to localized lattice distortion arising from the adatom. (i) Two divacancy defects, each having been transformedviatwo SW rotations, leading to a single isolated, rotated hexagon. Non-annotated images are presented inSupplementary Fig. S6. (j–l) Atomic models corresponding to the defect structures ing–i, respectively. Scale bars represent 1 nm. The colour scheme (dashed line annotations and model filling colour) denotes the number of carbons in the respective carbon ring, such that green, yellow, blue and dark blue represent 4-, 5-, 7- and 8-membered carbon rings, respectively. Full size image Figure 3: Defects created after 60 and 120 s exposures to the electron beam. ( a – c ) Annotated AC-TEM images of defects formed after 60 s of focussed electron beam irradiation. ( a ) Three linked divacancies. ( b ) A divacancy after a SW transformation. ( c ) Defects clustered around one of a pair of dislocations. Non-annotated images are presented in Supplementary Fig. S4 . ( d – f ) Atomic models of the defects presented in a – c , respectively. ( g – i ) Annotated AC-TEM images of defects formed after 120 s of focussed electron beam irradiation. ( g ) An enclosed, rotationally misaligned core of six hexagons, surrounded by a complete loop of pentagons and heptagons. ( h ) A larger, partially completed loop, isolating several rotated hexagons. A gap in the loop, filled by two hexagonal rings, is highlighted in red. The arrow marks an adatom, which inhibits direct interpretation of the area bordered in black due to localized lattice distortion arising from the adatom. ( i ) Two divacancy defects, each having been transformed via two SW rotations, leading to a single isolated, rotated hexagon. Non-annotated images are presented in Supplementary Fig. S6 . ( j – l ) Atomic models corresponding to the defect structures in g – i , respectively. Scale bars represent 1 nm. The colour scheme (dashed line annotations and model filling colour) denotes the number of carbons in the respective carbon ring, such that green, yellow, blue and dark blue represent 4-, 5-, 7- and 8-membered carbon rings, respectively. Full size image Figure 3 shows that extending the exposure time from 30 to 60 or 120 s resulted in the formation of larger defect structures. We show for 60 s three linked divacancies along the armchair direction ( Fig. 3a ), a divacancy plus a SW rotation ( Fig. 3b , similar to that shown in Fig. 2d ), and a complex defect structure along the zig–zag lattice direction, containing a dislocation pair and vacancies ( Fig. 3c ). Atomic models of the defect structures in Fig. 3a–c are presented in Fig. 3d–f , respectively. Further details of the atoms sputtered and bond rotations required to form these from a pristine lattice are included in supporting Supplementary Fig. S5 . Increasing the exposure to the focussed electron beam to 120 s allowed for the creation of defects of further complexity ( Fig. 3g–l ). Figure 3g shows six hexagons surrounded by a complete loop of pentagon–heptagon pairs. The central hexagons are rotationally misaligned by 30° with respect to the bulk graphene lattice, with the loop acting to screen this misaligned core from the rest of the lattice. Although this low-energy vacancy configuration has been hypothesized [22] , to the best of our knowledge this structure has not been directly observed before. Another set of rotationally misaligned hexagons are similarly enclosed in a nest of alternating pentagons and heptagons ( Fig. 3h ). However, in this image the structure of the loop is incomplete and two hexagons complete the circuit. Within a small area, denoted by the black border in Fig. 3h , it is difficult to clearly resolve the lattice structure to determine the bonding configuration due to the presence of an adatom (marked by an arrow), which is likely sorbed at the more reactive defect site [6] . The defects in Fig. 3g,h originate from multiple divacancy structures, akin to those illustrated by Fig. 3i . In this case two divacancy structures have each transformed through two SW rotations, leading to a single hexagon that is rotated by 30° with respect to the rest of the lattice. Several of these divacancy structures can form into the more complex configurations shown in Fig. 3g,h (ref. 22 ). Figure 3j–l presents atomic models of the defect structures in Fig. 3g–i , respectively. This ability to control the average complexity of defects created by adjusting the exposure time is summarized in Fig. 4 , which characterizes the defect structures directly after creation. 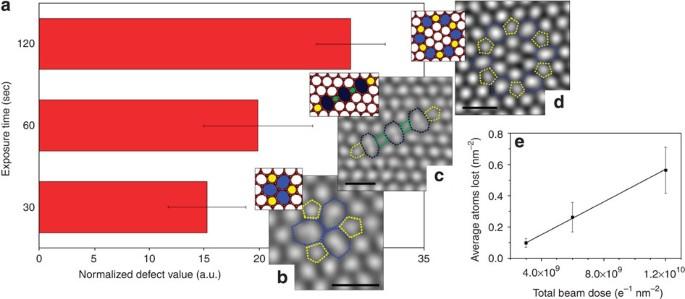Figure 4: Analysing the defect creation process. (a) A bar chart parameterizing the effect of exposure time on defect complexity, defined here as the number of non-six-membered carbon rings plus any rotationally mismatched six-membered rings in the irradiated area, parameterized as the NDV. Error bars are the calculated s.e. (b–d) Representative AC-TEM images for each exposure time (30, 60 and 120 s, respectively), along with an atomic model, (b) have a NDV of 6, (c) 7 and (d) 19 (7 rotated rings + 12 non-six-membered rings). The colour scheme (dashed line annotations and model filling colour) denotes the number of carbons in the respective carbon ring, such that green, yellow, blue and dark blue represent 4-, 5-, 7- and 8-membered carbon rings, respectively. Scale bars are 0.5 nm. (e) The average number of atoms lost per nm2as a function of total beam dose (e−1nm−2), yielding from the gradient a sputtering cross-section of 1.35×10−2barn. Error bars are the calculated s.e. NDV, normalized defect value. Figure 4e shows a linear plot of atoms lost per nm 2 as a function of total dose, the gradient of which we use to calculate a sputtering cross-section of 1.35×10 −2 barn. The complexity of the defects has been parameterized by assigning a value of one both to every non-six-membered ring and to rotationally misaligned six-membered rings present in the irradiated area (examples are shown in Supplementary Fig. S7 ). Exceptions to this are the isolated divacancies, which can freely oscillate between three stable configurations via SW rotations on a short-time scale, even under imaging doses ( Supplementary Fig. S8 ), and thus were assigned a value of 6. Representative annotated AC-TEM images, with accompanying atomic models, are also shown, with the complex closed loop structures only found at exposure times of 120 s. However, these longer exposure times do not guarantee the formation of these higher-level defects, but are a necessary prerequisite. Simpler single divacancy defects are still observed to form during some 120 s exposures. Exposure times beyond 120 s often led to holes opening up within the graphene sheet due to etching from impurities, hence the limit of 120 s exposure. We found that holes opened up even in regions of graphene that had not been directly exposed to the electron beam, but were close by and next to contamination. This indicates that the hole-opening process is not always driven by electron beam-induced sputtering and that an electron beam-mediated chemical etching method may not provide sufficient spatial control for defect creation. Figure 4: Analysing the defect creation process. ( a ) A bar chart parameterizing the effect of exposure time on defect complexity, defined here as the number of non-six-membered carbon rings plus any rotationally mismatched six-membered rings in the irradiated area, parameterized as the NDV. Error bars are the calculated s.e. ( b–d ) Representative AC-TEM images for each exposure time (30, 60 and 120 s, respectively), along with an atomic model, ( b ) have a NDV of 6, ( c ) 7 and ( d ) 19 (7 rotated rings + 12 non-six-membered rings). The colour scheme (dashed line annotations and model filling colour) denotes the number of carbons in the respective carbon ring, such that green, yellow, blue and dark blue represent 4-, 5-, 7- and 8-membered carbon rings, respectively. Scale bars are 0.5 nm. ( e ) The average number of atoms lost per nm 2 as a function of total beam dose ( e −1 nm −2 ), yielding from the gradient a sputtering cross-section of 1.35×10 −2 barn. Error bars are the calculated s.e. NDV, normalized defect value. Full size image Defect evolution and stability The stability of the defects created by irradiation was examined. 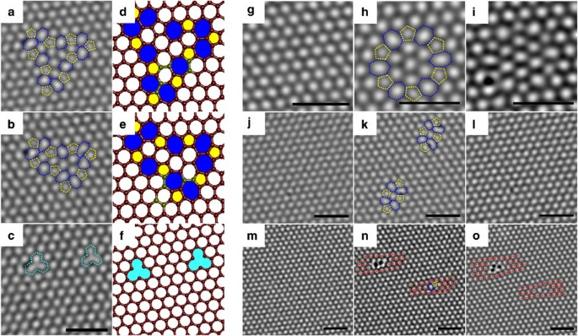Figure 5: The stability of created defects. (a–c) AC-TEM images and (d–f) accompanying atomic models, showing the near complete relaxation of a complex defect structure, observed under imaging BCD. After 360 s the structure changes to that shown inb; the atoms and bonds that undergo a Stone-Wales rotation are highlighted in gold ind, with resulting positions highlighted in gold ine. (c) The final image of the series, 660 s after initial observations, shows the defect reduced to two monovacancies (light blue, also highlighted inf). AC-TEM image (g) before and (h) after a 120-s high BCD exposure. (i) The same defect after 900 s of exposure to an imaging BCD, showing no change in configuration. (j) Pristine region of graphene lattice before focussed irradiation. (k) Two divacancy defects formed after 120 s high BCD exposure. (l) Quenching of the two divacancy defects back to pristine lattice after 480 s without irradiation (beam blanked). (m) Pristine graphene lattice before irradiation. (n) Creation of dislocations by 120-s exposure to high BCD irradiation. (o) Stability of two dislocation defects, with surrounding lattice planes highlighted in red, after 600 s without irradiation. Non-annotated AC-TEM images are presented inSupplementary Fig. S9. The colour scheme (dashed line annotations and model filling colour) denotes the number of carbons in the respective carbon ring, such that yellow and blue represent 5- and 7-membered carbon rings, respectively. Scale bars are 1 nm. Figure 5a–c shows the evolution and relaxation of a large defect configuration, shown earlier in Fig. 3g , to a near pristine lattice under normal imaging conditions. This defect configuration has been shown to have a low formation energy, and as such would be expected to be stable [22] . This is supported to a degree by our observations, where we were able to observe the defect for 6 min under imaging BCD conditions, before a set of three SW rotations (atoms and bonds that rotate are highlighted in gold in Fig. 5d ) causes it to collapse to an energetically less stable state. Over the course of a further 5 min of imaging the defect was observed to relax into a less disordered state, with the image series concluding with the defect reduced to two monovacancies in a graphene lattice. Given that the initial defect is formed from a combination of three divacancies, the presence of these residual vacancies is expected, and it is likely further observation would show the quenching of these residual monovacancies by additional mobile surface adatoms. Figure 5: The stability of created defects. ( a – c ) AC-TEM images and ( d – f ) accompanying atomic models, showing the near complete relaxation of a complex defect structure, observed under imaging BCD. After 360 s the structure changes to that shown in b ; the atoms and bonds that undergo a Stone-Wales rotation are highlighted in gold in d , with resulting positions highlighted in gold in e . ( c ) The final image of the series, 660 s after initial observations, shows the defect reduced to two monovacancies (light blue, also highlighted in f ). AC-TEM image ( g ) before and ( h ) after a 120-s high BCD exposure. ( i ) The same defect after 900 s of exposure to an imaging BCD, showing no change in configuration. ( j ) Pristine region of graphene lattice before focussed irradiation. ( k ) Two divacancy defects formed after 120 s high BCD exposure. ( l ) Quenching of the two divacancy defects back to pristine lattice after 480 s without irradiation (beam blanked). ( m ) Pristine graphene lattice before irradiation. ( n ) Creation of dislocations by 120-s exposure to high BCD irradiation. ( o ) Stability of two dislocation defects, with surrounding lattice planes highlighted in red, after 600 s without irradiation. Non-annotated AC-TEM images are presented in Supplementary Fig. S9 . The colour scheme (dashed line annotations and model filling colour) denotes the number of carbons in the respective carbon ring, such that yellow and blue represent 5- and 7-membered carbon rings, respectively. Scale bars are 1 nm. Full size image Although some defects relaxed to pristine graphene following exposure to the imaging beam, others were observed to be resilient to continued irradiation at a BCD ∼ 10 5 e − 1 nm −2 s −1 . Figure 5g–i shows a closed loop defect ( Supplementary Fig. S10 ) that was stable for a prolonged period of time under normal imaging conditions, with Fig. 5g before, Fig. 5h after 120 s of focussed irradiation and Fig. 5i after a further 780 s of imaging exposure. The defect did not change for over 900 s of exposure to imaging doses of irradiation. These defects, consisting of a closed loop of pentagon–heptagon pairs, have been proposed to occur intrinsically with low formation energies [28] . Kurasch et al . [29] showed that these closed-looped structures can unwind under higher BCDs of 10 7 e − 1 nm −2 s −1 . Divacancy defects were found to be less stable and susceptible to quenching by adatoms on the surface (see Supplementary Fig. S9 ). Figure 5j–l shows the creation of two divacancy defects by focussed irradiation from a pristine lattice. Following the recording of the image in Fig. 5k , the electron beam was blanked, preventing irradiation of the specimen, for 480 s. Subsequent images recorded from same region ( Fig. 5l ) showed the defects were quenched back to a pristine lattice, suggesting that defect annealing can occur in the absence of the electron beam. Created dislocations, such as the pair shown in Fig. 5m–o , were found to be predominantly stable against annihilation. From these observations we can conclude that quenching of simple divacancy defects can occur without electron beam irradiation. However, for the relaxation of more complex, closed-loop defects it is necessary to provide an initializing SW rotation to destabilize the defect, causing a cascade of further rotations culminating in a pristine lattice, with vacancy quenching also subsequently occurring in cases such as shown in Fig. 5c . The energy for this initializing SW rotation must come from the electron beam, as the thermal energy contribution alone is insufficient [30] , thus these defects are expected to remain stable when not subject to irradiation. The creation of vacancy defects at 80 kV, albeit under irradiation at higher BCD than normally used for imaging, implies that it is still possible to induce limited sputtering in graphene. Work conducted on an 80 kV AC-STEM system (see Supplementary Methods ) demonstrated that 80-kV electron beam irradiation of a single carbon atom at high doses of ∼ 2.54×10 10 e − 1 nm −2 s −1 , which is two orders of magnitude more than achieved using the focused TEM probe, does not lead to a sputtering event. This initially puzzling result suggests that the sub-threshold sputtering process does not depend on the dose received by a single carbon atom, but relies on an area of the sample to be irradiated. Chemical etching by surface contamination can be eliminated as the cause of the reported defects, as it does not produce defects at defined locations in a clean area of graphene, as demonstrated by AC-STEM data showing holes opening in the graphene areas away from the focus point of irradiation but near sources of iron contamination (see Supplementary Methods ). Furthermore, chemical etching typically produces holes rather than the defect structures observed here, with holes tending to appear for exposure times in excess of 120 s. Meyer et al . [31] studied the electron beam dependent cross-section for sputtering in graphene using a BCD of at most 10 6 e − 1 nm −2 s −1 , and at 80 kV they did not observe a single defect for a total dose of up to 10 10 e − 1 nm −2 . We measured a cross-section of 1.35×10 −2 barn for a BCD ∼ 10 8 e − 1 nm −2 s −1 , which is more than two orders of magnitude larger than the calculated value of 7×10 −5 barn reported in ref. 31 . This confirms that standard knock-on sputtering cannot be the mechanism in our observations. We discuss two possible explanations for the BCD-dependent cross-section within the irradiated area that are (i) lowering of the sputtering threshold due to weakening of the chemical bonds from ionization/plasmon excitations, or (ii) an increase in the out-of-plane atomic vibrations in graphene that provide additional momentum to enable an 80-keV electron to sputter a carbon atom. Calculations show that the threshold for sputtering has to be reduced by only ∼ 10% from 22 to 19.7 eV to achieve our experimentally observed cross-section (see Supplementary Discussion , Supplementary Fig. S12 ). We can discount electron beam-heating effects as graphene is an excellent thermal conductor; as such calculations show negligible overall temperature rise would be expected in our sample (see Supplementary Discussion , Supplementary Fig. S14 ) [32] , consistent with calculations on carbon nanotube heating [33] . Crucially, thermal conduction in graphene occurs via efficient phonon modes and a small contribution from free electrons [34] , [35] . Under continual irradiation there may be some depletion of electrons within the irradiated area, due to their involvement in thermal conduction, that could weaken the sp 2 bonds and lower the threshold for sputtering. However, given that the major contributor to thermal conduction in graphene arises from phonon propagation, it seems more likely that the excitation of phonon modes provides an increase in the out-of-plane velocity component that leads to our observed sputtering. Recent work has shown that flexural phonon modes have an essential role in thermal conductance in suspended graphene [36] . Graphene also has unusual and strong coupling between plasmons and phonons [37] , [38] . Thus, an inelastic collision may trigger a flexural phonon mode either directly or through plasmon coupling that causes a temporary increase in the out-of-plane motion of surrounding atoms, and if a subsequent elastic collision were to occur with one of these atoms then sputtering may result. For low BCDs, the probability of this occurring reduces because of the short lifetime of either the plasmon or phonon mode. The behaviour of flexural phonon modes in graphene follows a quadratic dispersion relationship and thus the density of states and its dependence on temperature are different to the Debye model [39] . Focussed electron beam irradiation may change the distribution of occupied phonon modes with an increased proportion of flexural modes at the expense of in-plane modes, while not changing the overall temperature of the system. Direct evidence of phonon excitations in graphene from electron beam irradiation has been reported in ref. 20 . Explanations of variations in the sputtering cross-section with BCD are known to be challenging, and further investigation is required to gain deeper insight into this phenomenon [32] . The ability to create defects in a controlled area, ( ∼ 10×10 nm 2 ), with variable complexity, opens up the possibility for enhanced engineering of graphene. The introduction of the focussed, high current density electron beam perturbs the system and leads to changes in the sputtering cross-section. Although we have observed that some structures simply revert back to a defect-free lattice, instances of beam-induced defects that are stable have also been observed. These latter, stable defects could provide the necessary reaction points for controlled functionalization, as they would likely be less susceptible to annealing during processing. We have shown that dislocation pairs known to induce strain in the lattice of graphene can be created by sputtering along the zig–zag lattice direction [40] . These results provide important foundations regarding which defects are stable enough to persist in graphene and thus be useful for future studies. CVD growth of graphene on liquid copper Graphene was synthesized by atmospheric pressure CVD, the complete details of synthesis and transfer are according to a previously reported method [41] . Graphene was grown on a molten copper sheet (Alfa Aesar, Puratonic 99.999% pure, 0.1 mm thick) of ∼ 1 cm 2 , resting on top of a similar-sized piece of molybdenum (Alfa Aesar, 99.95% pure, 0.1 mm thick). This was loaded into the quartz tube of the split-tube furnace CVD system, which was subsequently sealed, pumped to vacuum and backfilled with argon. Hundred standard cubic centimetres per minute (100 s.c.c.m.) H 2 /Ar (20% gas mix) and 200 s.c.c.m. pure Ar was flowed, and the furnace was ramped to 1,090 °C, whereupon the sample was slid into the furnace hot zone and annealed for 30 min, after which the CH 4 flow (1% gas mix in Ar) was enabled at 10 s.c.c.m. and the H 2 /Ar flow reduced from 100 to 80 s.c.c.m., while maintaining the pure argon gas line flow at 200 s.c.c.m. These conditions were maintained for 90 min to obtain continuous film growth. Following this the CH 4 flow was disabled and the sample immediately removed from the furnace hot zone, allowing for rapid cooling in the H 2 and Ar atmosphere. The sample was subsequently recovered from the quartz tube once sufficiently cool. Transfer A poly (methyl methacrylate) scaffold (8% wt. in anisole, 495 kDa molecular weight) was spin cast on to the graphene side of the graphene/copper/molybdenum sample at 4,700 r.p.m. for 60 s, and then cured at 180 °C for 90 s. The underlying molybdenum and copper were etched by floating the sample on an Fe(III)Cl 3 +HCl solution for several days, until just a transparent poly (methyl methacrylate)/graphene film remained suspended on the surface. This was thoroughly cleaned by transferring and floating onto clean deionized water several times, then transferred to a 30% HCl solution for 5 min, which was found to be critical to allow for thorough decontamination of the graphene and prevent iron-aided etching of the graphene ( Supplementary Methods ) [42] , [43] , rinsed again in DI water for 30 min [44] , and subsequently transferred to a holey silicon nitride TEM grid (Agar Scientific Y5385). Once left to dry for about an hour, the sample was baked on a hot plate at 150 °C for 15 min to remove water and greatly improve sample adhesion. Defect creation Defects were created at 2.5×10 6 magnification by focussing the beam to crossover on a region of graphene observed to be free of most contamination (a small quantity of amorphous carbon in the viewing area is desirable, as it is required for correcting the astigmatism of the beam). The beam profile is shown in Supplementary Fig. S1 , which is used to calculate an approximate BCD of BCD=1×10 8 e − 1 s −1 nm −2 . AC-TEM imaging The Oxford-JEOL JEM-2200MCO FEGTEM with CEOS hexapole aberration correctors, at an accelerating voltage of 80 kV, was used for electron beam irradiation and imaging. Image filtering techniques are described in Supplementary Methods . How to cite this article: Robertson, A.W. et al . Spatial control of defect creation in graphene at the nanoscale. Nat. Commun. 3:1144 doi: 10.1038/ncomms2141 (2012).